Klf5 controls bone marrow homing of stem cells and progenitors through Rab5-mediated β1/β2-integrin trafficking Krüppel-like factor 5 regulates pluripotent stem cell self-renewal, but its role in somatic stem cells is unknown. Here we show that Krüppel-like factor 5-deficient haematopoietic stem cells and progenitors fail to engraft after transplantation. This haematopoietic stem cell and progenitor defect is associated with impaired bone marrow homing and lodging and decreased retention in bone marrow, and with decreased adhesion to fibronectin and expression of membrane-bound β1/β2-integrins. In vivo -inducible gain-of-function of Krüppel-like factor 5 in haematopoietic stem cells increases haematopoietic stem cell and progenitor adhesion. The expression of Rab5 family members, mediators of β1/β2-integrin recycling in the early endosome, is decreased in Klf5 Δ/Δ haematopoietic stem cells and progenitors. Krüppel-like factor 5 binds directly to the promoter of Rab5a/b , and overexpression of Rab5b rescues the expression of activated β1/β2-integrins, adhesion and bone marrow homing of Klf5 Δ/Δ haematopoietic stem cells and progenitors. Altogether, these data indicate that Krüppel-like factor 5 is indispensable for adhesion, homing, lodging and retention of haematopoietic stem cells and progenitors in the bone marrow through Rab5-dependent post-translational regulation of β1/β2 integrins. Krüppel-like factor 5 (Klf5) is a member of the Klf family of transcription factors. Klf5 is expressed in highly proliferative epithelial cell types during embryogenesis and in the adult including the skin, gut, prostate, lung, mammary gland and bladder, as well as in immortalized epithelial cell lines and proliferating primary cultures [1] . Mice null for the Klf5 alleles are embryonic lethal and die before embryonic day 8.5 (ref. 2 ). Klf5 works as a downstream activator of transcriptional programs associated with pluripotent stem cell activity and differentiation [2] , and its deficiency results in impaired blastocyst formation and implantation [3] . Using in vivo models, Klf5 has been shown to have a role in biological processes such as embryonic development, cardiovascular remodelling, adipogenesis, inflammatory stress responses, and intestinal and lung development [4] . However, our understanding of the specific roles of Klf5 in adult stem cells from high-turnover tissues is minimal. Haematopoietic stem cells (HSCs) located in the bone marrow (BM) represent an example of self-renewing cells, which need to replenish billions of cells a day. BM HSCs are located within specialized BM niches where they recognize specific adhesion ligands that are present on cells and on the extracellular matrix. Modulation of HSC adhesion influences essential cellular processes which are required for homing and engraftment, a crucial process that allows HSC to be transplanted in the clinical setting. Major molecular mediators of these effects are the integrins, heterodimeric transmembrane glycoproteins that link extracellular matrix components to the intracellular actin cytoskeleton. Integrins consist of α- and β-subunits that act together to bind specific ligands. At present, 8 α- and 18 β-integrin subunits have been described. Of these, the β1-subunit, a component in 11 receptors with distinct chains [5] , has been shown to be crucial in the function of HSC [6] , [7] . Upon ligand binding, the short cytoplasmic sequence of all integrin variants regulates several types of transmembrane signalling events [8] . Biochemical recycling assays have clearly demonstrated that certain integrin heterodimers are continually internalized from the plasma membrane into endosomal compartments and then recycled back to the cell surface, thus completing an endo-exocytic cycle [9] . Recycling of heterodimers containing β1-integrins has been shown to be crucial to the control of cell adhesion [10] by controlling the levels of active and inactive β1-integrin on the cell membrane [11] . Active endosome trafficking ensures spatio-temporal regulation of the turnover of adhesion complexes at both the trailing and leading edges of a polarized migrating cell. This involves enhanced internalization within early endosomes and recycling at the leading and trailing edges coupled with localized Rac guanosine triphosphatase (GTPase)-dependent organization of the actin cytoskeleton, and increased focal adhesion assembly/disassembly rates. The Rab family of small GTPases regulates the membrane trafficking and intracellular vesicle transport, including receptor-mediated endocytosis, exocytosis and receptor recycling [12] . Aberrant expression of the Rab GTPases has been found in many human diseases including cancer [13] . The Rab5 subfamily members, Rab5a and Rab5b, are mainly located at the cytosolic face of the plasma membrane, early endosomes, and clathrin-coated vesicles. They have been shown to be key regulators of intracellular vesicle traffic from the plasma membrane to early endosomes [14] , and their activity is required for maturation of the β1-integrin-containing early endosomes [15] . In this report, we demonstrate that Klf5 is required for the adhesion, homing and engraftment of HSC. Loss of Klf5 results in decreased membrane expression of active membrane β1- and β2-integrin in HSC and progenitor (HSC/P) cells, but does not result in defective primary or stressed hematopoiesis. The reduced expression of membrane β1/β2-integrins on the membrane of HSC/P depends upon Klf5-mediated expression of Rab5. Klf5 is required for hematopoietic repopulation To understand the role of Klf5 in HSC/P activity, we crossed Klf5 flox/flox mice [4] and Mx-Cre transgenic [16] mice to generate Mx1-Cre;Klf5 flox/flox mice, and then administered polyinositide:polycytidine (pI:pC) to induce Mx1-Cre expression and in vivo deletion of floxed Klf5 alleles. Peripheral blood genotyping and expression of Klf5 mRNA and protein in HSC/P demonstrated efficient gene deletion when compared with Mx1-Cre;Klf5 +/+ wild type (WT) mice ( Fig. 1a–c ) or Mx1-Cre;Klf5 flox/flox without pl:pC injection as controls ( Supplementary Fig. S1 ). To examine whether the specific loss of Klf5 expression in HSC/P impairs the blood-formation ability of Klf5-deficient mice, peripheral blood was collected at different time points after the last pI:pC injection ( Supplementary Fig. S2a ), and the numbers of circulating myeloid, T cells and B cells in peripheral blood at 15 and 44 days post pI:pC administration were counted. In agreement with the described role of Klf5 in granulocyte-macrophage differentiation in response to G-CSF signalling [17] , [18] , Klf5 Δ/Δ mice showed a modest decrease in the myeloid cell count, without T- or B-cell lymphopenia ( Supplementary Fig. S2b ), thrombocytopenia or reticulocytopenia (Day 0 data in Supplementary Fig. S3d,e ). BM HSC/P content was also normal in Klf5-deficient mice as analyzed for as long as 6 weeks after the last pI:pC injection ( Supplementary Fig. S2c ). 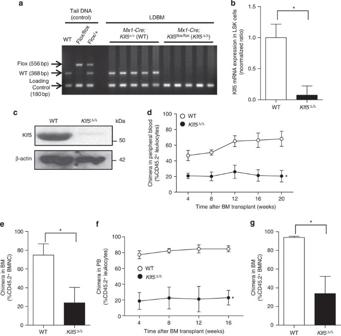Figure 1: Klf5 deficiency impairs HSC competitive repopulation capacity. (a) PCR genotyping of WT, floxed andKlf5Δ/Δalleles from tail and low-density BM (LDBM) cell genomic DNA isolated from the BM of Mx1-Cre; WT or Mx1-Cre;Klf5Δ/Δmice after five pI:pC injections administered every other day. (b) mRNA expression (Q-RT–PCR) analysis ofKlf5in LSK cells isolated from pI:pC-treated Mx1-Cre, WT or Mx1-Cre andKlf5Δ/Δmice. Data are presented as mean±s.d., *P=0.0002, Studentt-test. (c) Immunoblot for Klf5 protein expression in Lin/c-kit-/Sca-1- (LSK) BM cells from pI:pC-treated Mx-Cre;WT or Mx1-Cre;Klf5Δ/Δmice. (d) Competitive repopulation assay to determine the role of Klf5 in HSC engraftment. Lethally irradiated primary recipient CD45.1+mice were transplanted with a mixture of 3 × 106Mx1-Cre;Klf5Δ/ΔBM cells (CD45.2+) and 3 × 106WT BM CD45.1+cells (solid circles). The control group was transplanted with a mixture of 3 × 106Mx1-Cre; WT BM cells (CD45.2+) and 3 × 106WT BM CD45.1+cells (open circles). Data are presented as mean±s.d., *P=0.019, Studentt-test. (e) Chimera analysis of the BM of primary recipients at 20 weeks after transplantation. Data are presented as mean±s.d., *P<0.0001, Studentt-test. (f) Peripheral blood (PB) chimera of secondary recipients transplanted with 10 × 106BM cells obtained from primary mice (ind). Data are presented as mean±s.d., *P=0.008, analysis of variance (ANOVA) test. (g) BM chimera in secondary recipients after 4 months of transplantation. *P=0.001, Studentt-test. (b,d–g) Eight to sixteen mice per group were transplanted and analyzed in two independent experiments. Data are presented as mean±s.d. BMNC, BM nucleated cell. Figure 1: Klf5 deficiency impairs HSC competitive repopulation capacity. ( a ) PCR genotyping of WT, floxed and Klf5 Δ/Δ alleles from tail and low-density BM (LDBM) cell genomic DNA isolated from the BM of Mx1-Cre; WT or Mx1-Cre; Klf5 Δ/Δ mice after five pI:pC injections administered every other day. ( b ) mRNA expression (Q-RT–PCR) analysis of Klf5 in LSK cells isolated from pI:pC-treated Mx1-Cre, WT or Mx1-Cre and Klf5 Δ/Δ mice. Data are presented as mean±s.d., * P =0.0002, Student t -test. ( c ) Immunoblot for Klf5 protein expression in Lin/c-kit-/Sca-1- (LSK) BM cells from pI:pC-treated Mx-Cre;WT or Mx1-Cre; Klf5 Δ/Δ mice. ( d ) Competitive repopulation assay to determine the role of Klf5 in HSC engraftment. Lethally irradiated primary recipient CD45.1 + mice were transplanted with a mixture of 3 × 10 6 Mx1-Cre; Klf5 Δ/Δ BM cells (CD45.2 + ) and 3 × 10 6 WT BM CD45.1 + cells (solid circles). The control group was transplanted with a mixture of 3 × 10 6 Mx1-Cre; WT BM cells (CD45.2 + ) and 3 × 10 6 WT BM CD45.1 + cells (open circles). Data are presented as mean±s.d., * P =0.019, Student t -test. ( e ) Chimera analysis of the BM of primary recipients at 20 weeks after transplantation. Data are presented as mean±s.d., * P <0.0001, Student t -test. ( f ) Peripheral blood (PB) chimera of secondary recipients transplanted with 10 × 10 6 BM cells obtained from primary mice (in d ). Data are presented as mean±s.d., * P =0.008, analysis of variance (ANOVA) test. ( g ) BM chimera in secondary recipients after 4 months of transplantation. * P =0.001, Student t -test. ( b , d – g ) Eight to sixteen mice per group were transplanted and analyzed in two independent experiments. Data are presented as mean±s.d. BMNC, BM nucleated cell. Full size image Klf5 regulates cell proliferation and survival in other tissues, such as the basal layer of the oesophagus or the intestinal crypts [19] , [20] . Klf5 deficiency had no effect on proliferation or survival of HSC/P as assayed by in vivo bromodeoxyuridine incorporation or caspase-3 assay, respectively ( Supplementary Fig. S3a,b ). To assess whether the loss of Klf5 altered the hematopoietic ability of HSC/P function dependent on Klf5 activity under stress conditions, Klf5-deficient and WT mice were injected with 5-fluorouracil, a sublethal cytostatic drug that only spares quiescent HSC and induces stress recovery hematopoiesis in surviving HSC that are forced to enter the cell cycle. Interestingly, we observed no significant recovery impairment in the peripheral blood counts of neutrophils ( Supplementary Fig. S3c ), platelets ( Supplementary Fig. S3d ), or reticulocytes ( Supplementary Fig. S3e ), supporting the concept that Klf5 is dispensable in the regulation of HSC/P-dependent stress-induced hematopoiesis. Competitive repopulation is the gold standard assay for HSC regenerative activity where a small population of HSC compete against normal HSC to repopulate a full animal. In this assay, intravenously transplanted HSC compete for lodging sites within the BM niches, and fit HSC engraft in a complex process that involves cellular and extracellular matrix adhesion and migration towards chemo-attractant gradients. The contribution of the different HSC/P populations to engraftment is monitored by analyzing the hematopoietic chimera populations in the peripheral blood and BM at different time points. Serial transplantation of competitively transplanted animals provides specific information on long-term engrafting HSC populations. Transplantation of Klf5 Δ/Δ HSC/P into lethally irradiated recipients revealed abnormal competitive engraftment and hematopoiesis at each test interval for peripheral blood ( Fig. 1d ) and BM ( Fig. 1e ), suggesting that all Klf5 Δ/Δ HSC/P populations were similarly impaired in their ability to contribute to repopulation in vivo . This phenotype was also reproduced in serially transplanted secondary recipient mice ( Fig. 1f ), indicating that the repopulation ability of the long-term HSC (LT-HSC) compartment was impaired. The impaired engraftment of Klf5-deficient HSC did not induce significant bias or skew in multi-lineage repopulation. Myeloid, B and T cells behaved similarly to the overall leukocyte engraftment in primary and secondary recipients ( Supplementary Fig. S4a–f ). These data indicate that Klf5 in HSC/P is dispensable for basal and stressed hematopoietic activity, but indispensable for competitive engraftment of HSC/P. Klf5 Δ/Δ HSC/P have decreased adhesion and lodging in BM Because proliferation and survival of Klf5 Δ/Δ HSC/P was not impaired, we next examined whether the impaired competitive repopulation ability of Klf5 Δ/Δ HSC/P was accompanied by changes in their homing to the BM. An equal number of WT or Klf5 Δ/Δ BM cells were injected into non-irradiated WT littermates. Quantitative phenotypic and functional analysis of the homing of HSC/P was performed using flow-cytometry analysis of 5-(and-6)-carboxyfluorescein diacetate succinimidyl ester (CFSE)-labelled BM cells or a clonogenic progenitor assay (colony-forming unit cells (CFU-C)). At 16 h after transplantation, femoral BM cells from recipient mice were collected and assayed. The homing of different populations (LT-HSC, short-term HSC (ST-HSC), multipotential progenitors (MPP) and CFU-C) of Klf5 Δ/Δ HSC/P was significantly impaired at similar levels (~50–70% reduction, Fig. 2a–d , Supplementary Fig. S5 ). Specific locations within the BM cavity are associated with enrichment of HSC niches [21] , [22] . To evaluate homing to these HSC-niche enriched BM areas, we analyzed the HSC/P lodging in serial femoral longitudinal sections of mice transplanted with CFSE-labelled WT or Klf5-deficient Lin − /c-kit + /Sca-1 + (LSK) cells, as previously described [23] , [24] . Lodging of LSK cells ( Fig. 2e ) within the putative microanatomical endosteal space of the BM ( Fig. 2e ) was significantly impaired. About 45% of WT HSC/P lodged in the endosteal region, whereas only 9% of the Klf5-deficient HSC/P that homed to the BM were found inside the endosteal area ( P <0.05) ( Fig. 2g ). The deficient BM homing/lodging of transplanted HSC/P was also associated with a ~3.5-fold increase in circulating HSC/P ( Fig. 2h ), while the number of HSC/P in the BM was the same in both WT and Klf5-deficient mice ( Supplementary Fig. S2c ). Together, these data indicate that the retention of Klf5 Δ/Δ HSC/P in BM is decreased. 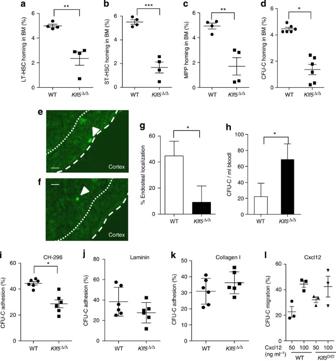Figure 2:Klf5Δ/ΔHSC/P are impaired in their lodging and adhesion to fibronectin. (a–d) Homing of HSC/P in the BM of WT orKlf5Δ/Δmice at 16 h post transplantation.n=4 to 6 mice per group. (a) Homing of CFSE-labelled LT-HSC (defined as Lin−/c-kit+/Sca1+/CD34−/CD135−BM cells), **P=0.0033, Studentt-test. (b) Homing of CFSE-labelled ST-HSC (defined as Lin−/c-kit+/Sca1+/CD34+/CD135−BM cells). ***P=0.0003, Studentt-test. (c) Homing of CFSE-labelled multipotential progenitors (MPPs, defined as Lin−/c-kit+/Sca1+/CD34+/CD135+BM cells). **P=0.0047, Studentt-test. (e,f) Illustration in longitudinal femoral sections of how endosteal localization (e) and central localization (f) were defined for location of transplanted CFSE+LSK BM cells. Short arrows define specific fluorescent cells. Dashed lines indicate the endosteum layer that separates the bone cortex from the BM. Endosteal area was defined as the area covered by 12 cell diameters perpendicular to the endosteum (bidirectional arrow, space between dashed line and dotted line). Central area was defined as the one beyond the endosteal area. Scale bar, 20 μm. (g) Percentage of CFSE+LSK BM WT versusKlf5Δ/Δfound in the endosteal area. *P=0.04, Studentt-test,n=56 per group. (h) PB count of CFU-C in primary WT andKlf5Δ/Δmice. *P=0.013, Studentt-test,n=9 per group. (i–k) Adhesion of WT andKlf5Δ/ΔBM CFU-C to the recombinant fibronectin fragment CH-296, *P=0.007, Studentt-test,n=6 per group (i), laminin (j) and collagen I (k). (l) Chemotaxis of WT andKlf5Δ/ΔBM CFU-C to Cxcl12,n=3 per group. Figure 2: Klf5 Δ/Δ HSC/P are impaired in their lodging and adhesion to fibronectin. ( a – d ) Homing of HSC/P in the BM of WT or Klf5 Δ/Δ mice at 16 h post transplantation. n =4 to 6 mice per group. ( a ) Homing of CFSE-labelled LT-HSC (defined as Lin − /c-kit + /Sca1 + /CD34 − /CD135 − BM cells), ** P =0.0033, Student t- test. ( b ) Homing of CFSE-labelled ST-HSC (defined as Lin − /c-kit + /Sca1 + /CD34 + /CD135 − BM cells). *** P =0.0003, Student t -test. ( c ) Homing of CFSE-labelled multipotential progenitors (MPPs, defined as Lin − /c-kit + /Sca1 + /CD34 + /CD135 + BM cells). ** P =0.0047, Student t -test. ( e , f ) Illustration in longitudinal femoral sections of how endosteal localization ( e ) and central localization ( f ) were defined for location of transplanted CFSE + LSK BM cells. Short arrows define specific fluorescent cells. Dashed lines indicate the endosteum layer that separates the bone cortex from the BM. Endosteal area was defined as the area covered by 12 cell diameters perpendicular to the endosteum (bidirectional arrow, space between dashed line and dotted line). Central area was defined as the one beyond the endosteal area. Scale bar, 20 μm. ( g ) Percentage of CFSE + LSK BM WT versus Klf5 Δ/Δ found in the endosteal area. * P =0.04, Student t -test, n =56 per group. ( h ) PB count of CFU-C in primary WT and Klf5 Δ/Δ mice. * P =0.013, Student t -test, n =9 per group. ( i – k ) Adhesion of WT and Klf5 Δ/Δ BM CFU-C to the recombinant fibronectin fragment CH-296, * P =0.007, Student t -test, n =6 per group ( i ), laminin ( j ) and collagen I ( k ). ( l ) Chemotaxis of WT and Klf5 Δ/Δ BM CFU-C to Cxcl12, n =3 per group. Full size image HSC/P adhesion and retention within the BM largely depend on their binding ability to key proteins, components of the extracellular matrix. Among them, binding to fibronectin and laminin has been postulated to be crucial in the control of HSC adhesion to BM niches [25] , [26] . During HSC engraftment, fibronectin binds to heterodimers formed by β1-integrins [27] , and laminin binds to heterodimers containing β1- and β3-integrin chains [25] . We found that the adhesion of Klf5 Δ/Δ HSC/P to CH-296, a C-terminus fibronectin peptide, was significantly decreased compared with WT HSC/P ( Fig. 2i ). In contrast, the adhesion ability of Klf5 Δ/Δ HSC/P to laminin ( Fig. 2j ) or collagen type I ( Fig. 2k ), which bind to multiple partner receptors including different β-integrin chains [28] , was not significantly impaired. The chemokine Cxcl12 is a crucial molecule that mediates the retention and homing of HSC/P [29] , [30] . The migration of Klf5-deficient HSC/P towards a Cxcl12 gradient ( Fig. 2l ) was not significantly impaired, regardless the tested concentration (50–100 ng ml −1 ). These findings indicate that the deletion of Klf5 in HSC/P impairs their ability to engraft BM and is associated with defects in BM homing/lodging and fibronectin adhesion. Klf5 gain-of-function increases adhesion to fibronectin To delineate whether Klf5 expression regulates the adhesion of HSC/P, we crossed stem cell leukaemia ( Scl ) promoter-driven tetracycline transactivator ( Scl-tTA ) transgenic mice [31] with transgenic animals expressing Klf5 driven by a tetracycline responsive element (TRE) [32] to generate Scl-tTA/TRE-Klf5 mice. In this murine model, Klf5 overexpression is induced after doxycycline withdrawal and is restricted to HSC and early progenitors expressing the transcriptional factor Scl [16] . Serial protein-expression analysis from Scl-tTA/TRE-Klf5 mice demonstrated a peak of Klf5 expression in LSK BM cells by day +5 after doxycycline withdrawal (tet-off) ( Fig. 3a ), which was confirmed by immunoblotting of sorted BM LSK cells ( Supplementary Fig. S1 ). Quantitative PCR with reverse transcription (Q-RT–PCR) of LSK BM cells showed a fivefold increase in the levels of Klf5 mRNA by the same day ( Fig. 3b ). Overexpression of Klf5 was associated with increased (~50%) adhesion of LSK BM cells to fibronectin ( Fig. 3c ), whereas their migratory ability towards Cxcl12 was not significantly changed ( Fig. 3d ). The homing of Klf5-overexpressing HSC was not significantly improved ( Fig. 3e ), suggesting functional saturation of in vivo homing. Altogether, the results of loss-of-function and gain-of-function of Klf5 expression indicated that Klf5 regulates the adhesion of HSC/P to fibronectin. 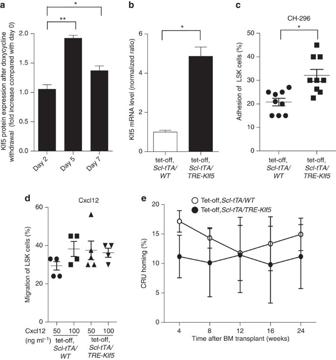Figure 3: Inducible expression of Klf5in vivoinduces increased adhesion to fibronectin and normal BM homing. (a,b) Klf5 expression in LSK BM cells isolated from tet-off,Scl-tTA/WT(WT) orScl-tTA/TRE-Klf5mice. (a) Protein was measured by intracellular flow cytometry on BM LSK cells fromScl-tTA/TRE-Klf5mice collected on days 2, 5 and 7 post doxycycline withdrawal.N=3 independent animals per group. Data represent mean±s.e.m. **P=0.001, ***P=0.0006, Studentt-test. (b) mRNA on sorted BM LSK cells after 5 days post doxycycline withdrawal. ***P=0.0002, Studentt-test. (c) Adhesion of LSK BM cells to fibronectin from tet-off,WTorScl-tTA/Tre-Klf5mice. *P=0.019, Studentt-test. (d) Chemotaxis of LSK BM cells to CXCL12 from tet-off,WTorScl-tTA/Tre-Klf5mice. Data are presented as mean±s.d. (e) Homing of WT and Klf5-overexpressing HSC. Graph depicts the homing (%) after 3 h post transplantation of competitive repopulation units (CRU) analyzed as engrafting units after co-transplantation with CD45.1+competitor BM cells into congenic recipients, analyzed at 4, 8, 12, 16 and 24 weeks post transplantation.N=8 to 10 mice per group, from two independent experiments. Figure 3: Inducible expression of Klf5 in vivo induces increased adhesion to fibronectin and normal BM homing. ( a , b ) Klf5 expression in LSK BM cells isolated from tet-off, Scl-tTA/WT (WT) or Scl-tTA/TRE-Klf5 mice. ( a ) Protein was measured by intracellular flow cytometry on BM LSK cells from Scl-tTA/TRE-Klf5 mice collected on days 2, 5 and 7 post doxycycline withdrawal. N =3 independent animals per group. Data represent mean±s.e.m. ** P =0.001, *** P =0.0006, Student t -test. ( b ) mRNA on sorted BM LSK cells after 5 days post doxycycline withdrawal. *** P =0.0002, Student t -test. ( c ) Adhesion of LSK BM cells to fibronectin from tet-off, WT or Scl-tTA/Tre-Klf5 mice. * P =0.019, Student t -test. ( d ) Chemotaxis of LSK BM cells to CXCL12 from tet-off, WT or Scl-tTA/Tre-Klf5 mice. Data are presented as mean±s.d. ( e ) Homing of WT and Klf5-overexpressing HSC. Graph depicts the homing (%) after 3 h post transplantation of competitive repopulation units (CRU) analyzed as engrafting units after co-transplantation with CD45.1 + competitor BM cells into congenic recipients, analyzed at 4, 8, 12, 16 and 24 weeks post transplantation. N =8 to 10 mice per group, from two independent experiments. Full size image Klf5 regulates the localization of β1-/β2-integrins in HSC/P Based on the data supporting a role for Klf5 in BM HSC/P homing and fibronectin-mediated adhesion, we hypothesized that Klf5 may control β-integrin function. To understand whether the expression of β integrins was affected by Klf5 expression, we analyzed the cell-membrane expression of β1-, β2-, β3-, β7-integrin and two major alpha chain partners in HSC/P, α4- and α5-integrin, and the homing cell-adhesion molecule, which also binds to the fibronectin fragment CH-294. β1-integrin has been reported to be essential for HSC/P homing through binding to fibronectin [33] , [34] , while β2-integrin expression has a minimal role in HSC homing [35] . β3 and β7 integrin chains, also expressed in HSC/P, are not well characterized functionally in relation to HSC/P homing. We found that the membrane expression of β1- and β2-integrins was significantly decreased in Klf5-deficient LSK BM cells compared with their WT counterparts ( Fig. 4a , P =0.025, Student t -test). The expression levels of membrane α4-, α5-, β3- or β7-integrins were, however, not significantly changed ( Supplementary Fig. S6a,b ). Interestingly, HSC/P whole-cell lysate immunoblots showed upregulation of the overall cellular level of β1- or β2-integrin protein expression ( Fig. 4b ). Scl-tTA/TRE-Klf5 transgenic expression in BM HSC/P resulted in the opposite phenotype of Klf5 Δ/Δ HSC/P and was associated with increased membrane expression of β1-and β2-integrin, but not other integrin chains ( Fig. 4c and Supplementary Fig. S6c ), indicating the existence of a positive correlation between the expression level of Klf5, membrane β1- and β2-integrin and adhesion to fibronectin. Consistent with the post-translational nature of the changes in β1-/β2-integrin expression, mRNA levels of Klf5-deficient and Klf5-overexpressing mice were not affected by the level of expression of Klf5 compared with their control counterparts ( Supplementary Fig. S6d ). In agreement, with the absence of difference in Cxcl12-directed migration, we found that the expression level of Cxcl12 receptor, Cxcr4, in HSC/P was not affected by the expression of Klf5. Its levels in Klf5-deficient or Scl-tTA/TRE-Klf5 HSC/P, were comparable to those in WT HSC/P ( Supplementary Fig. S6e,f ). These results suggest that Klf5 specifically controls the localization of β1- and β2-integrins on the cell membrane. 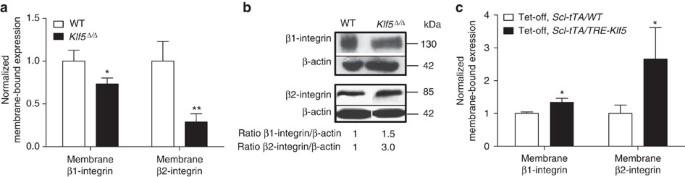Figure 4: DefectiveKlf5Δ/ΔHSC/P homing is attributed to a post-translational decrease in membrane-bound β1- and β2-integrins. (a) Expression of membrane β1- and β2-integrin in WT (empty bars) andKlf5Δ/Δ(solid bars) LSK BM cells as assessed by flow cytometry (normalized mean fluorescence intensity ratio). *P=0.03, **P=0.004, Studentt-test,n=3 to 4 per group. (b) Representative example of immunoblot of β1- and β2-integrin expression of whole-cell lysates from WT andKlf5Δ/ΔLSK BM cells. Densitometric ratio analysis was calculated. (c) Expression of membrane β1- and β2-integrin in LSK BM cells from tet-off,Scl-tTA/WT(empty bars) orScl-tTA/TRE-Klf5mice (solid bars). *P=0.01, Studentt-test,n=4 per group. Figure 4: Defective Klf5 Δ/Δ HSC/P homing is attributed to a post-translational decrease in membrane-bound β1- and β2-integrins. ( a ) Expression of membrane β1- and β2-integrin in WT (empty bars) and Klf5 Δ/Δ (solid bars) LSK BM cells as assessed by flow cytometry (normalized mean fluorescence intensity ratio). * P =0.03, ** P =0.004, Student t -test, n =3 to 4 per group. ( b ) Representative example of immunoblot of β1- and β2-integrin expression of whole-cell lysates from WT and Klf5 Δ/Δ LSK BM cells. Densitometric ratio analysis was calculated. ( c ) Expression of membrane β1- and β2-integrin in LSK BM cells from tet-off, Scl-tTA/WT (empty bars) or Scl-tTA/TRE-Klf5 mice (solid bars). * P =0.01, Student t -test, n =4 per group. Full size image Klf5 controls the expression of Rab5 mRNA in HSC/P To identify direct Klf5 targets involved in adhesion activity and expression of β1- and β2-integrin on the cell membrane, we performed gene-expression profiling using cDNA from RNA isolated from WT or Klf5 Δ/Δ HSC/P (Gene Expression Omnibus (GEO) accession number GSE43806 ). Of the 1,146 genes that showed significant differential expression, gene ontology analysis identified 14 major functional subgroups ( Supplementary Fig. S7a ). The expression of other Klf genes was not significantly modified by Klf5 deficiency ( Supplementary Table S1 ), and Ingenuity analysis identified regulation of two groups of genes responsible for gene processes as statistically significant ( Supplementary Table S2 ). A search for downregulated genes with known activity on integrin transport identified several members of the Rab GTPase family, including Rab5b , Rab17 , Rab19 and the downstream Rab3 effector Rph3a . Rab proteins are small GTPases that are involved in the traffic of endocytosis vesicles, control the endosomal traffic of β-integrins [29] and control cell adhesion [30] . Although Rab3 and Rab19 are associated with the process of general trans-Golgi or post-Golgi transport [36] , Rab5 and Rab17 have a specific role in controlling the formation of early endosomes and, therefore, endosomal traffic [37] , [38] , an essential in β-integrin recycling [39] . We hypothesized that HSC/P Klf5 could transcriptionally regulate the expression of Rab5 and/or Rab17, thereby regulating β1- and β2-integrin trafficking from the cell membrane. Q-RT–PCR analysis showed that Klf5 regulates Rab5a/b expression in both Klf5 Δ/Δ (~50% reduction) and Scl-tTA/TRE-Klf5 transgenic HSC/P ( Fig. 5a , Supplementary Fig. S7b ), but Q-RT–PCR did not confirm downregulated expression of Rab17 mRNA expression in Klf5-deficient HSC/P ( Supplementary Fig. S7c ). Decreased Rab5a/b mRNA expression in Klf5-deficient HSC/P was associated with decreased Rab5a/b protein expression, which also decreased ~50% ( Fig. 5c ). We identified the putative Klf5-binding sites (CACCC- and GC-rich motif) in the promoter region of Rab5a and Rab5b . Chromatin immunoprecipitation analysis revealed that Klf5 binds to upstream sequences near the transcription start site of both Rab5a and Rab5b loci in BM HSC/P ( Fig. 5d ). Taken together, these results suggest that Rab5a and Rab5b genes are direct transcriptional targets of Klf5. 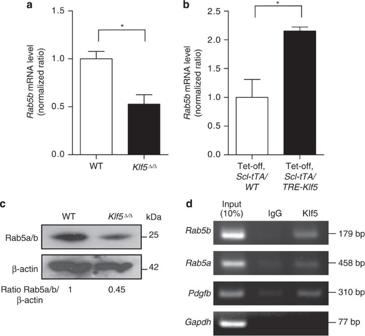Figure 5: Klf5 directly regulates the expression of Rab5 family proteins. (a,b)n=3 per group;Rab5bexpression (Q-RT–PCR) of LSK BM cells from WT andKlf5Δ/Δmice (a) or tet-off,Scl-tTA/WTandScl-tTA/TRE-Klf5mice. *P=0.028, Studentt-test. (b) Data are presented as mean±s.d. (*P=0.033, Studentt-test,n=3 mice per group). (c) Representative example of immunoblotting of Rab5a/b in WT andKlf5Δ/ΔLSK BM cells.N=3 mice per group. (d) Chromatin immunoprecipitation analysis on lysates from Lin−BM cells. Following the immunoprecipitation using Klf5-specific antibody, PCR was performed using primers designed to encompass the putative Klf5-binding site in the proximal promoter region. Amplification of aPdgfbgenomic region serves as positive control. Immunoprecipitation using IgG and amplification of theGapdhgene serve as negative controls. Figure 5: Klf5 directly regulates the expression of Rab5 family proteins. ( a , b ) n =3 per group; Rab5b expression (Q-RT–PCR) of LSK BM cells from WT and Klf5 Δ/Δ mice ( a ) or tet-off, Scl-tTA/WT and Scl-tTA/TRE-Klf5 mice. * P =0.028, Student t -test. ( b ) Data are presented as mean±s.d. (* P =0.033, Student t -test, n =3 mice per group). ( c ) Representative example of immunoblotting of Rab5a/b in WT and Klf5 Δ/Δ LSK BM cells. N =3 mice per group. ( d ) Chromatin immunoprecipitation analysis on lysates from Lin − BM cells. Following the immunoprecipitation using Klf5-specific antibody, PCR was performed using primers designed to encompass the putative Klf5-binding site in the proximal promoter region. Amplification of a Pdgfb genomic region serves as positive control. Immunoprecipitation using IgG and amplification of the Gapdh gene serve as negative controls. Full size image Overexpressed Rab5b rescues Klf5-dependent HSC/P activity Cell homing requires regulated turnover of adhesions, which can be achieved by a combination of integrin activation and inactivation at the cell surface and dynamic cell-surface targeting and endocytic removal of activated integrins from the plasma membrane [40] , [41] . We hypothesized that Rab5 controls the levels of active β1- and β2-integrin on the membrane, and that the deficient homing of Klf5 Δ/Δ HSC/P was a result of their inability to express active β1-integrin on the membrane, available to bind fibronectin. If true, the exogenous expression of Rab5b in Klf5 Δ/Δ HSC/P should rescue the expression of both membrane-bound active β1- and β2-integrins, and revert the adhesion and homing defects. For this purpose, we performed rescue experiments of adhesion and homing of HSC/P isolated from Vav1-Cre/Klf5 flox/flox mice where Vav1 -promoter-driven Cre expression restricts the deficiency of Klf5 to hematopoietic cells [42] . These mice are viable, have a normal lifespan and their HSC/P completely lack Klf5 protein expression (hematopoietic Klf5 Δ/Δ , H- Klf5 Δ/Δ , Fig. 6a ). H- Klf5 Δ/Δ LSK BM cells were lentivirally transduced with bicistronic vectors expressing either Rab5b and enhanced green fluorescent protein (EGFP) (Rab5b) or only EGFP (Mock). Q-RT–PCR confirmed the complete loss of Klf5 transcript expression in H- Klf5 Δ/Δ HSC/P and the presence of exogenous Rab5b expression in Rab5b-transduced cells ( Supplementary Fig. S7d,e ). Immunofluorescence analysis by both flow-cytometry and confocal microscopy analysis of β1-integrin expression on the membrane of EGFP + HSC/P showed that exogenous expression of Rab5b rescued total membrane β1-integrin expression ( Fig. 6b ), and especially membrane-bound active β1-integrin expression ( Fig. 6d–g ), but did not significantly modify the levels of inactive membrane β1-integrin ( Supplementary Fig. S8a–d ). Similarly, membrane β2-integrin expression was also rescued by exogeneous expression of Rab5b ( Fig. 7a–d ), suggesting that restoration of membrane expression of active β1- and β2-integrin depend on Rab5 expression. 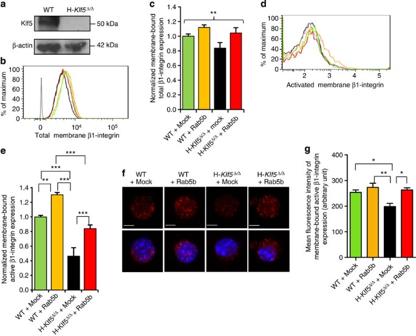Figure 6: Lentiviral-vector-mediated Rab5b expression rescues the total and activated fraction of membrane-bound β1-integrin in Klf5Δ/ΔHSC/P. (a) Immunoblotting of Klf5 in LSK isolated fromVav1-Cre-WT(WT) orVav1-Cre-Klf5flox/floxmice(H-Klf5Δ/Δ). β-actin shown in figure as a loading control. (b–e) Fluorocytometric analysis of membrane-bound integrin expression of mock- or Rab5b-transduced LSK BM cells from WT orH- Klf5Δ/Δmice. Sorted LSK BM cells were transduced with a lentiviral vector expressing Rab5b and eGFP or eGFP only (Mock) as a control WT-Mock (green line or bar), WT-Rab5b (orange line or bar),H-Klf5Δ/Δ-Mock (black line or bar) andH-Klf5Δ/Δ-Rab5b (red line or bar) LSK BM cells. (b,c) Membrane expression of total β1-integrin. (b) Representative example of flow-cytometry analysis; (c) normalized membrane-bound total β1-integrin expression (n=3 replicates per group). **P=0.0042, analysis of variance (ANOVA test). (d,e) Membrane expression of activated β1-integrin. (d) Representative example of flow-cytometry analysis. (e) Normalized membrane-bound activated β1-integrin expression (n=3 replicates per group). (f,g) Confocal microscopy analysis of membrane expression of activated β1-integrin. (f) Representative picture of membrane-bound active β1-integrin. Active β1-integrin (red) and 4′,6-diamidino-2-phenylindole (DAPI; blue, overlaid in lower row pictures). Scale bar, 5 μm. (g) Mean fluorescence intensity of membrane-bound active β1-integrin expression as analyzed by confocal microscopy. A minimum of 50 cells per group was analyzed by confocal microscopy. (e,g) Data are presented as mean±s.e.m., *P<0.05, **P<0.01, ***P<0.001. ANOVA test with Bonferroni correction. Figure 6: Lentiviral-vector-mediated Rab5b expression rescues the total and activated fraction of membrane-bound β1-integrin in Klf5 Δ/Δ HSC/P. ( a ) Immunoblotting of Klf5 in LSK isolated from Vav1-Cre-WT (WT) or Vav1-Cre-Klf5 flox/flox mice ( H-Klf5 Δ/Δ ). β-actin shown in figure as a loading control. ( b – e ) Fluorocytometric analysis of membrane-bound integrin expression of mock- or Rab5b-transduced LSK BM cells from WT or H- Klf5 Δ/Δ mice. Sorted LSK BM cells were transduced with a lentiviral vector expressing Rab5b and eGFP or eGFP only (Mock) as a control WT-Mock (green line or bar), WT-Rab5b (orange line or bar), H-Klf5 Δ/Δ -Mock (black line or bar) and H-Klf5 Δ/Δ -Rab5b (red line or bar) LSK BM cells. ( b , c ) Membrane expression of total β1-integrin. ( b ) Representative example of flow-cytometry analysis; ( c ) normalized membrane-bound total β1-integrin expression ( n =3 replicates per group). ** P =0.0042, analysis of variance (ANOVA test). ( d , e ) Membrane expression of activated β1-integrin. ( d ) Representative example of flow-cytometry analysis. ( e ) Normalized membrane-bound activated β1-integrin expression ( n =3 replicates per group). ( f , g ) Confocal microscopy analysis of membrane expression of activated β1-integrin. ( f ) Representative picture of membrane-bound active β1-integrin. Active β1-integrin (red) and 4′,6-diamidino-2-phenylindole (DAPI; blue, overlaid in lower row pictures). Scale bar, 5 μm. ( g ) Mean fluorescence intensity of membrane-bound active β1-integrin expression as analyzed by confocal microscopy. A minimum of 50 cells per group was analyzed by confocal microscopy. ( e , g ) Data are presented as mean±s.e.m., * P <0.05, ** P <0.01, *** P <0.001. ANOVA test with Bonferroni correction. 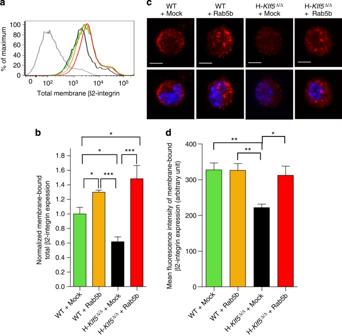Figure 7: Lentiviral-vector-mediated Rab5b expression rescues the membrane-bound β2-integrin expression in Klf5Δ/ΔHSC/P. (a–d) Membrane expression of β2-integrin. (a) Representative example of flow-cytometry analysis. (b) Normalized membrane-bound total β2-integrin expression analyzed by flow cytometry. Data are presented as mean±s.e.m. (n=3 replicates per group). (c) Representative example of membrane expression of membrane β2-integrin (red) analyzed by confocal microscopy. 4′,6-diamidino-2-phenylindole (DAPI, blue, overlaid in lower row pictures) was used for nuclear counterstain. Scale bar, 5 μm. (d) Mean fluorescence intensity of membrane-bound β2-integrin expression as analyzed by confocal microscopy. A minimum of 50 cells per group was analyzed by confocal microscopy. Data are presented as mean±s.e.m., *P=0.05, **P=0.01, ***P=0.01, ANOVA test with Bonferroni correction. Full size image Figure 7: Lentiviral-vector-mediated Rab5b expression rescues the membrane-bound β2-integrin expression in Klf5 Δ/Δ HSC/P. ( a – d ) Membrane expression of β2-integrin. ( a ) Representative example of flow-cytometry analysis. ( b ) Normalized membrane-bound total β2-integrin expression analyzed by flow cytometry. Data are presented as mean±s.e.m. ( n =3 replicates per group). ( c ) Representative example of membrane expression of membrane β2-integrin (red) analyzed by confocal microscopy. 4′,6-diamidino-2-phenylindole (DAPI, blue, overlaid in lower row pictures) was used for nuclear counterstain. Scale bar, 5 μm. ( d ) Mean fluorescence intensity of membrane-bound β2-integrin expression as analyzed by confocal microscopy. A minimum of 50 cells per group was analyzed by confocal microscopy. Data are presented as mean±s.e.m., * P =0.05, ** P =0.01, *** P =0.01, ANOVA test with Bonferroni correction. Full size image Functionally, the exogenous expression of Rab5b rescued the impaired adhesion of H- Klf5 Δ/Δ HSC/P to fibronectin, but unlike the overexpression of Klf5 ( Fig. 3c ), the overexpression of Rab5b did not increase the adhesion of WT HSC/P to fibronectin ( Fig. 8a ). Finally, the overexpression of Rab5b in H- Klf5 Δ/Δ HSC/P restored their ability to home to the BM to the same level as WT HSC/P ( Fig. 8b ). These results indicate that HSC/P BM homing activity is dependent on direct Klf5 transcriptional control of Rab5 expression, which mediates active β1-integrin expression on the cell membrane and subsequent HSC/P adhesion to the BM microenvironment. 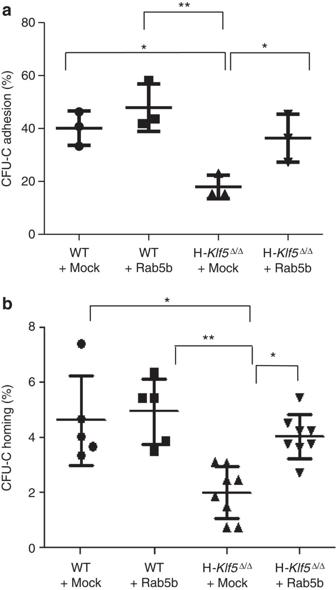Figure 8: Forced Rab5b expression rescues the impaired adhesion and homing defect of hematopoietic-specificKlf5Δ/ΔHSC/P. (a) Adhesion to fibronectin ofH-Klf5Δ/ΔLSK cells was rescued by exogenous expression of Rab5b (n=3 per group, in each of two independent experiments). (b) CFU-C homing in the BM ofH-Klf5Δ/Δmice was rescued by lentivirus transduction of Rab5b. Homing was analyzed at 16 h after transplantation (similar toFig. 2a–d). Data are presented as mean±s.d.n=5 to 8 mice per group; *P<0.05, **P<0.01, ***P<0.001, ANOVA test with Bonferroni correction. Figure 8: Forced Rab5b expression rescues the impaired adhesion and homing defect of hematopoietic-specific Klf5 Δ/Δ HSC/P. ( a ) Adhesion to fibronectin of H-Klf5 Δ/Δ LSK cells was rescued by exogenous expression of Rab5b ( n =3 per group, in each of two independent experiments). ( b ) CFU-C homing in the BM of H-Klf5 Δ/Δ mice was rescued by lentivirus transduction of Rab5b. Homing was analyzed at 16 h after transplantation (similar to Fig. 2a–d ). Data are presented as mean±s.d. n =5 to 8 mice per group; * P <0.05, ** P <0.01, *** P <0.001, ANOVA test with Bonferroni correction. Full size image The Klf transcriptional factor family has both essential and redundant functions. Klf5, similar to the other 16 members of the Klf family, contains three zinc-finger domains that function in DNA binding. In hematopoiesis, Klf proteins have been shown to have redundant roles. For instance, Klf1- and Klf2-dependent globin-expression regulation have been shown to compensate each other in primitive erythtopoiesis, and Klf1 has a distinct role in the expression of β-globin in definitive erythropoiesis [43] . Klf2, Klf4 and Klf5 have redundant roles in a circuitry controlling embryonic stem cell pluripotency [44] . Klf5 is highly expressed in HSCs and differentiated myeloid cells [45] . Klf5 expression, controlled by Klf4, appears to control the granulocyte-macrophage differentiation of committed myeloid progenitors/precursors in response to granulocyte colony-stimulating factor signalling [17] , [18] and to regulate monocyte/macrophage differentiation and activation [46] , [47] . In embryonic stem cells, the Klf family members Klf2, Klf4 and Klf5 have redundant roles in self-renewal regulation [44] , and Klf5 is required to prevent differentiation [48] . However, the specific roles of Klf5 in postnatal stem cell activity remain to be determined. We report a previously unknown role for Klf5 in BM adhesion, retention, homing, endosteal lodging and engraftment of HSC/P. Although Klf5 is not essential for HSC self-renewal, Klf5 is an essential transcriptional factor controlling BM homing, lodging in the endosteal space, engraftment and BM retention of HSC/P. Using gene-expression profiling validated by Q-RT–PCR in WT or Klf5 Δ/Δ HSC/P, we identified several members of the Rab GTPase family, including Rab5a, Rab5b and Rab17 as downstream targets of Klf5. Of these, transcriptional regulation of Rab5 was demonstrated, and protein levels and chromosome immunoprecipitation confirmed that Klf5 binds Rab5a and Rab5 proximal promoters in HSC/P. Klf5-downstream targets in other stem cells such as embryonic stem cells do not include Rab5 genes [49] , strongly suggesting that the cellular context of transcriptional co-activators is crucial in target selection. Rab5 function is essential for endosomal traffic [37] , [38] , which is essential for β-integrin recycling [39] . Decreased expression of Rab5 proteins interferes with the membrane localization of heterodimers containing β1- and β2-integrins (but not α-integrin chains or CD44), which results in defective adhesion of HSC/P to fibronectin. Inducible overexpression of Klf5 in HSC results in the opposite effect by increasing the membrane expression of β1- and β2-integrins and adhesion to the relevant extracellular matrix protein fibronectin [26] . However, Klf5 overexpression does not result in increased BM homing ability over WT HSC/P, suggesting that Klf5-mediated responses are saturated at baseline in vivo . Exogenous expression of Rab5b corrects the membrane localization of activated β1- and β2-integrins, the HSC/P adhesion to fibronectin, and in vivo BM homing, which is associated with decreased adhesion to fibronectin and in vivo BM homing of Klf5-deficient HSC/P. Our work indicates that Klf5 is a positive regulator of the lodging of HSC/P within the BM niches through the regulation of Rab5-dependent integrin recycling. Although other Klf genes may partly replace Klf5, we observed no apparent compensatory transcriptional regulation of other Klf genes in HSC/P. Our findings underscore the importance of the binding of β1- and β2-integrins containing heterodimers to functionally active HSC niches within the BM [6] , such as those that require fibronectin adhesion [27] . Under steady-state conditions, that is, when HSC/P are firmly adherent to the BM stroma, cells express multiple integrins, however, the main integrin determinants of steady-state HSC/P adhesion to the BM stroma are the α4β1- and α5β1-integrins, whose counter receptors are either fibronectin or the cell-surface ligand, VCAM-1. In fact, α4-integrin expression is essential for HSC/P adhesion and is different in BM HSC/P compared with circulating HSC/P [50] . A deficiency of one or more β-chains can be compensated by the formation of heterodimers with alternative β-chains like β3-integrins, which are also expressed by HSC [51] . The conformation of integrins, and thus their ability to bind to extracellular matrix proteins, is modulated by the interaction of their cytoplasmic domain with intracellular signalling and cytoskeletal proteins. Outside-in activation of integrins results from a conformational change upon ligand binding. Activation involves severing a salt bridge that tethers the cytoplasmic domains of the α- and β-chains and conformational rearrangement of the A domain of the β-chain to form a high-affinity matrix-binding pocket, bringing the integrin into the fully active state [52] . A general feature of activated integrin traffic is that, rather than degradation, they undergo internalization and are subsequently recycled back to the cell surface [9] . Up to 50% of activated integrins on the cell surface are recycled back to the membrane. Both internalization and recycling rates are accelerated by Rab proteins. The specificity of integrin-Rab protein binding has been shown in mutational analysis of the cytosolic domain of the β1-integrin heterodimers, which mediates interaction with the early endosomal Rab proteins Rab5 and Rab17 (ref. 38 ). The process of integrin internalization and recycling ensures spatio-temporal regulation of the activated integrin complex turnover at both the trailing and leading edges of a polarized cell upon adhesion to the extracellular matrix. Activated integrins are continuously transported to a pericentriolar/juxtanuclear recycling compartment using the clathrin/Rab5/Rab11 endosome system. As the earliest endosome-interacting Rab, Rab5 protein has key roles in both cell adhesion and motility through the regulation of β1-integrin recycling [53] . A reduction of as little as 50% in the levels of Rab5 proteins is sufficient to abrogate cellular endocytosis [54] . Although Rab5-GTP is the active form, the phenotype induced by Klf5 deficiency seems to respond to a decrease in the expression of Rab5 genes, because overexpression of Rab5b rescues integrin expression on the membrane, adhesion to fibronectin and BM homing of HSC/P. Mechanistically, Rab5 activity has been shown to be independent of phophoinositide 3-kinase and the small GTPases, Ras, Rho and Cdc42 (ref. 55 ) and to be dependent on Rac1 activation downstream [56] , which is required for HSC homing [24] . Our data indicate that Rab5 deficiency induced by loss of the transcriptional factor Klf5 results in the loss of membrane-bound expression of β1- and β2-integrins, including the active form of β1-integrin, and results in decreased adhesion to the extracellular matrix and homing and lodging in the BM endosteal space. Altogether, our data indicate that Klf5 has an essential role in the transcriptional regulation of Rab5 expression, which in turn controls β1- and β2-integrin availability and localization within the membrane, and HSC/P adhesion and homing within specific BM HSC/P niches. Animal models All the animals were backcrossed for a minimum of five generations into C57Bl/6 background. For inducible Klf5 gene inactivation in the hematopoietic compartment, Mx1-Cre mice [16] were crossed with Klf5 flox/flox mice [4] ( Klf5 Δ/Δ ). Klf5 deletion was induced by intraperitoneal administration of double-stranded RNA pI:pC (Amersham Pharmacia Biotech, Germany) (200 μg) every other day for a total of five times. Experiments were performed after a minimum of 7 days after the last pI:pC injection. For constitutive Klf5 gene inactivation, Vav1-Cre mice [42] were crossed with Klf5 flox/flox mice. For inducible Klf5 overexpression in HSC/P, Scl-tTA transgenic mice [31] were crossed with TRE-Klf5 mice [32] . BM was analyzed on day +5 post doxycycline withdrawal. HSC competitive repopulation assay Adult recipient mice were lethally irradiated (7+4.75 Gy, split doses at a dose rate of 58–63 cGy min −1 ; separated by 3 h, and previously demonstrated to eliminate all endogenous BM CFU-C) [24] . For competitive repopulation experiments, 3 × 10 6 CD45.2 + BM nucleated cells were mixed with 3 × 10 6 CD45.1 + BM nucleated cells and were transplanted into lethally irradiated CD45.1+ B6.SJLPtprca Pep3b/BoyJ recipient mice. ST-HSC and LT-HSC engraftment was analyzed in peripheral blood at 4-week intervals and on week 20 in the BM, to analyze the contribution of CD45.2+ leukocyte chimera and lineage differentiation by flow-cytometry analysis. Homing assays WT or Klf5 Δ/Δ animals were killed, and single cell suspensions of the BM from the lower limbs and pelvis were prepared and used for transplantation. BM cells (2 × 10 4 ) were plated in methylcellulose culture media (MethoCult; Stem Cell Technologies, Vancouver, BC, Canada) for CFU-C assay to quantify the initial content of hematopoietic progenitors. Ten million BM donor cells were injected through the tail vein into lethally irradiated C57Bl/6 recipient mice. Sixteen hours after transplant, the recipient mice were killed and the BM cells of the lower limbs and pelvis were collected and cultured in triplicate for CFU-C assay. Homing of immunophenotypically identified HSC/P was performed as previously published [57] , Briefly, 20 × 10 6 low-density WT or Klf5-deficient BM cells were labelled with 5μM CFSE (Molecular Probes, Life Technologies, Grand Island, NY). Cells were labelled for analysis of LT-HSC, defined as Lin − /c-kit + /Sca1 + /CD34 (RAM34) − /CD135 (4G8) −, ST-HSC, defined as Lin − /c-kit + /Sca1 + /CD34 + /CD135 − and multipotential progenitor, defined as Lin − /c-kit + /Sca1 + /CD34 + /CD135 + BM cells, before and 16 h after infusion into congenic myeloablated animals. For homing of transduced HSCs/Ps, 1 × 10 3 sorted LSK cells (WT+Mock, WT+Rab5b, Klf5 Δ/Δ +Mock or Klf5 Δ/Δ +Rab5b) were plated in methylcellulose culture media for CFU-C assay to quantify the initial content of hematopoietic progenitors. Sorted LSK donor cells (1 × 10 4 ) were injected through the tail vein into lethally irradiated C57Bl/6 recipient mice. Sixteen hours after transplant, the recipient mice were killed and the BM cells of the lower limbs and pelvis were collected and cultured in triplicate for CFU-C assay. To estimate the BM recovery, the femora, tibiae and pelvis were considered to contain 25% of the overall BM [58] . For Klf5-overexpressing HSC homing assay, 2.5 × 10 8 BM cells from tet-off, Scl-tTA/WT (WT) or Scl-tTA/TRE-Klf5 mice were injected through the tail vein into lethally irradiated (7+4.75 Gy) C57Bl/6 recipient mice. Three hours after transplant, the recipient mice were killed and the BM cells of the lower limbs and pelvis were collected. The BM cells (CD45.2 + ) were then transplanted into lethally irradiated CD45.1 + B6.SJLPtprca Pep3b/BoyJ recipient mice together with 5 × 10 5 CD45.1 + BM cells, and followed by competitive repopulation assay. ST-HSC and LT-HSC engraftment was analyzed in peripheral blood drawn at 4, 8, 12, 15 and 24 weeks post transplantation for the contribution of CD45.2+ leukocytes. Competitive repopulating units were calculated as previously described [59] , [60] . BM spatial distribution assay It was performed as previously described [23] , [24] . Briefly, sorted LSK cells were stained with 5 μM CFSE (Molecular Probes, Life Technologies). A total of 4 × 10 5 CFSE + cells were injected intravenously in non-conditioned C57Bl/6 recipients. After 16 h, mice were killed by terminal pentobarbital anaesthesia (30 mg kg −1 intraperitoneally), their hearts were cannulated through their left ventricles and a systemic perfusion of PBS/2% paraformaldehyde/0.05% glutaraldehyde was initiated at 4 ml min −1 for 15 min. Subsequently, femorae were removed, and after 2–3 weeks of incubation in 10% EDTA, pH 7.4 for decalcification, they were subsequently dehydrated in graded ethanol and embedded in paraffin. Longitudinal sections (4 μm) of each femur were cut, dewaxed and rehydrated. Every other longitudinal section (up to 20 sections per femur) was washed in PBS before mounting in Pro-Long Gold Antifade Reagent (Invitrogen, Life Technologies) and used for analysis. All sections were analyzed under an epifluorescent microscope (AxioObserver Z1; Zeiss, Gottingen, Germany) using a fluorescein isothiocyanate filter for specific signal and a rhodamine filter to discriminate autofluorescence. Analysis was performed by counting 56 sections, with a minimum of three mice per group. Endosteal area was defined as the area covered by 12 cell diameters perpendicular to the endosteum. Adhesion and migration assays Adhesion of HSC/P was performed by incubating 5 × 10 4 low-density BM (LDBM) cells from WT or Klf5 Δ/Δ mice onto a recombinant human fibronectin fragment CH-296 (RetroNectin; Takara Bio Inc., Japan), laminin (Invitrogen) or collagen type I (Life Technologies) for 1 h. An aliquot of LDBM cells was set aside for CFU-C assay to calculate the number of input cells. Non-adherent cells were removed carefully by washing in PBS at least twice, and the adherent cells retrieved by trypsinization. The percentage of adhesion was calculated from the input and output cell assay results. To assay adhesion using Scl-tTA/TRE-Klf5 mice, input and output cells were stained with LSK markers, and the percentage of the LSK cell population was analyzed by flow cytometry. Migration of HSC/P was analyzed by incubating 5 × 10 4 LDBM cells derived from WT or Klf5 Δ/Δ animals, on the top chamber of a 24-well transwell plate (Corning Inc., Lowell, MA). Recombinant Cxcl12 (50 or 100 ng ml −1 ; R&D Systems, Inc., Minneapolis, MN) was placed in the bottom wells, and the 24-well plate was incubated at 37 °C, 5% CO 2 . After 4 h of incubation, cells from the bottom chamber were collected by tripsinization, washed in PBS and the number of migrated hematopoietic progenitors was determined by CFU-C assay. The percentage of migrating cells was determined dividing the number of colonies present in the output fraction by the total number of input CFU-C. Input and output CFU-C were analyzed in triplicate. For migration assays using HSC/P Klf5-overexpressing mice, LSK BM cells were counted before and after migration. Confocal microscopy immunoflouorescence analysis For immunofluorescence analysis by confocal microscopy of membrane integrin expression on transduced HSC/P, LSK BM cells from VavCre;Wt and VavCre;Klf5 Δ/Δ mice were sorted and transduced with mock or Rab5b lentiviral vectors, and then allowed to adhered to the poly- L -lysine-coated slides. The adhered cells were fixed with 4% paraformaldehyde in PBS for 30 min and then blocked with 5% normal mouse serum. Cells were treated with primary antibody against the active form of β1 integrin (9EG7) or inactive form of β1 integrin (MAB13) or with Rat anti mouse β2 integrin antibody (C71/16), followed by treatment with Alexa-Fluor 568-conjugated goat anti-Rat IgG and Topro3 for nuclear staining. Cells were mounted with Vectashield mounting media containing antifading agent (Vector Labs, Burlingame, CA). The stained cells were analyzed by LSM 510 confocal system (Carl Zeiss) equipped with an inverted microscope (Observer Z1; Carl Zeiss) using Plan Apochromat 63 × 1.4 NA oil immersion lense. Argon ion 488, HeNe543 and HeNe633 laser lines were used to excite EGFP, Alexa Fluor568 and ToPro3, respectively. The emission signals were collected using band pass filters BP 505–530 for EGFP, BP 560–615 for Alexa Fluor568 and a long pass filter 650LP for ToPro3. Confocal images through optical plane along the z axis from top to bottom of cells were acquired at a resolution of 512 × 512 pixels with a bit depth of 12 bits. Images were acquired using Zen2009 imaging software (Carl Zeiss). To present the β1- or β2-integrin staining throughout the cell surfaces, the composite image of all the optical plane along the z axis of the cell was generated using Zen2009 software. The mean fluorescence intensities of the secondary antibody for active β1-integrin, inactive β1-integrin and β2 integrin on three-dimensional reconstituted cells were measured using Imaris Bitplane software. A minimum of 50 cells was analyzed per group and anti-integrin staining. Lentiviral Rab5b transduction The lentiviral vector pCDH-MCS-EF1-copGFP carrying the sequence of Klf5 was used to produce the virus. The empty vector was used as negative control. LSK BM cells (1 × 10 5 cells per sample) were cultured in IMDM, 10% FCS, 100 IU penicillin, 0.1 mg ml −1 streptomycin, 100 ng ml −1 stem cell factor and 50 ng ml −1 thrombopoietin and lentiviral supernatant (two rounds separated 16 h, multiplicity of infection=20) for 48 h at 37 °C and either sorted for EGFP expression or analyzed by flow cytometry. Statistical analysis Student t -test or analysis of variance followed by Bonferroni correction was used for statistical significance test. Level of significance was established at 0.05. Additional methods and any associated references are available in Supplementary Information . How to cite this article: Ishikawa, E. T. et al . Klf5 controls bone marrow homing of stem cells and progenitors through Rab5-mediated β1/β2-integrin trafficking. Nat. Commun. 4:1660 doi: 10.1038/ncomms2645 (2013).